Growth dynamics and gas transport mechanism of nanobubbles in graphene liquid cells Formation, evolution and vanishing of bubbles are common phenomena in nature, which can be easily observed in boiling or falling water, carbonated drinks, gas-forming electrochemical reactions and so on. However, the morphology and the growth dynamics of the bubbles at nanoscale have not been fully investigated owing to the lack of proper imaging tools that can visualize nanoscale objects in the liquid phase. Here, we demonstrate for the first time that the nanobubbles in water encapsulated by graphene membrane can be visualized by in-situ ultra-high vacuum transmission electron microscopy. Our microscopic results indicate two distinct growth mechanisms of merging nanobubbles and the existence of a critical radius of nanobubbles that determines the unusually long stability of nanobubbles. Interestingly, the gas transport through ultrathin water membranes at nanobubble interface is free from dissolution, which is clearly different from conventional gas transport that includes condensation, transmission and evaporation. Nanoscale bubbles are related to various important biological and chemical phenomena [1] , [2] . There have been intensive efforts to characterize the nanobubbles in liquid phase [3] , [4] , [5] , [6] , [7] , [8] , [9] , [10] , which includes ion conductance measurement through a solid-state nanopore [11] , topographic imaging by atomic force microscopy (AFM) [12] and direct visualization by optical methods [13] , [14] . None of these, however, is capable of imaging the liquid-phase nanobubbles in real time with sub-10 nm resolution. In this regard, in-situ transmission electron microscopy (TEM) [15] , [16] would be the best method to observe the behaviours of nanobubbles, but the resolution is still limited by the thickness and the robustness of liquid cell membranes. Recently, it was reported that graphene can be utilized as a perfect liquid cell membrane for in-situ TEM imaging of nanocrystal growth thanks to its atomic thickness, flexibility, extraordinary mechanical strength and high conductivity [17] . Here, we tried to investigate the evolution of nanobubbles by encapsulating them in a graphene liquid cell membrane for in-situ TEM imaging in ultra-high vacuum (UHV-TEM). Observation of nanobubbles The graphene liquid cell was fabricated by the sequential wet transfer of monolayer graphene synthesized by chemical vapour deposition ( Supplementary Fig. 1 ) [18] , [19] , [20] . The water islands are naturally captured during the wet transfer process of graphene to a graphene-supported TEM grid ( Supplementary Fig. 2 ). As shown in Fig. 1 , the top and side views of nanobubbles show the plano-convex morphology whose diameter ranges from 5 to 15 nm. It should be noted that the high mechanical flexibility and strength of graphene allows the cross-sectional imaging of nanobubbles in a folded (or cut) liquid cell ( Supplementary Fig. 3 ). Even though the image resolution in side views is not high enough to confirm the exact shapes of all the nanobubbles, the majority of the observed bubbles shows a plano-convex shape whose contact angle varies from 60 to 90° ( Fig. 1e–g and Supplementary Figs 4 and 5 ). This range of contact angles was used to calculate the internal pressure of nanobubbles using Young-Laplace equation, Δ P =2 γ / R c , where Δ P is the pressure difference across the nanobubble interface, γ is the surface tension of water and R c is the curvature radius of nanobubbles ( Fig. 1h ). For example, Young-Laplace pressure inside a 10-nm-diameter nanobubble, which has a contact angle of 72°, is calculated to be 27 MPa, which is 270 times higher than ambient pressure. 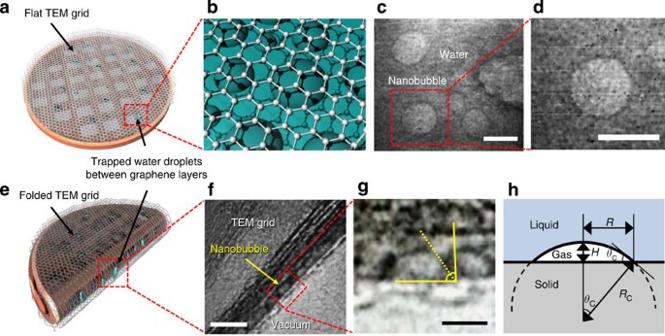Figure 1: Morphology of nanobubbles in graphene liquid cell. (a–d) A graphene liquid cell fabricated on a flat TEM grid (copper or molybdenum) showing the top views of nanobubbles. (candd)In-situsnapshot images of nanobubbles obtained by ultra-high vacuum (UHV) TEM (200 keV, ~5 × 10−9Torr). Scale bars, 10 nm. (e–g) A folded graphene liquid cell showing the side views of nanobubbles. The contact angles were roughly measured to be 60°–90°. Scale bars forfandg, 10 and 5 nm, respectively. (h) The schematic image of a nanobubble on solid surface and its structural parameters including surface radius (R), contact angle (θC), curvature radius (RC) and height (H). The full movie is available inSupplementary Movie 1. Figure 1: Morphology of nanobubbles in graphene liquid cell. ( a – d ) A graphene liquid cell fabricated on a flat TEM grid (copper or molybdenum) showing the top views of nanobubbles. ( c and d ) In-situ snapshot images of nanobubbles obtained by ultra-high vacuum (UHV) TEM (200 keV, ~5 × 10 −9 Torr). Scale bars, 10 nm. ( e – g ) A folded graphene liquid cell showing the side views of nanobubbles. The contact angles were roughly measured to be 60°–90°. Scale bars for f and g , 10 and 5 nm, respectively. ( h ) The schematic image of a nanobubble on solid surface and its structural parameters including surface radius ( R ), contact angle ( θ C ), curvature radius ( R C ) and height ( H ). The full movie is available in Supplementary Movie 1 . Full size image Stability of nanobubble According to classical diffusion theory, the lifetime of a nanobubble was predicted to be ~1 μs (ref. 21 ). In fact, however, nanobubbles are very stable even for several hours as revealed by liquid-phase AFM [22] . Many explanations on this superstability of nanobubbles were proposed, including stabilization by three-phase contact line pinning [23] and dynamic equilibrium at water–vapour interface [24] , [25] . In addition, the critical radius of stable nanobubbles was predicted to be ~1.7 nm by molecular dynamic simulation [26] and ~85 nm by dynamic equilibrium theory [25] , but there has been no experimental confirmation so far. Here we show, for the first time, that the critical radius of stable nanobubbles is 6.3±0.8 nm as shown in Fig. 2a,b . For the nanobubble radius below the critical radius, the radius keeps decreasing until it completely collapses, whereas the nanobubble lager than 6.3±0.8 nm persists for more than 10 min. The model calculation based on the structural parameters from the TEM observation gives the stable radii range of 5.04–5.21 nm for the contact angle range of 60°–90° ( Supplementary Fig. 6 ), which falls into the critical radii range of vanishing and stable nanobubbles in Fig. 3a,b , even though the attraction between the gas molecule and graphene surface can be neglected in our model ( Supplementary Notes ). 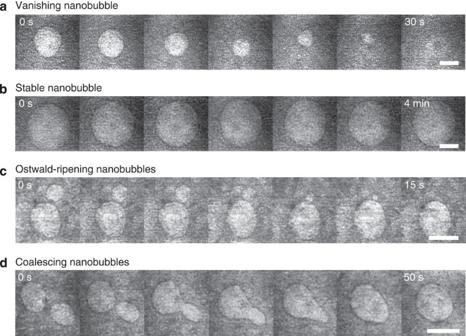Figure 2: Time evolution of different kinds of single and double nanobubbles. (a,b) The snap shots of TEM images showing the vanishing and stable nanobubbles, respectively. The nanobubbles smaller than critical radius tend to shrink with time and disappear in ~40 s, whereas the larger bubbles persist for more than 10 min. Scale bars, 5 nm. The full movie is available inSupplementary Movie 2. (c,d) The snap shots of TEM images showing the merging of adjacent two nanobubbles observed for 15 and 50 s, respectively. When the nanobubble sizes are significantly different, it shows an Ostwald ripening-like merging process, whereas the similar-sized bubbles are coalescing as their inter-bubble boundary breaks. Scale bars, 10 nm. The full movie is available inSupplementary Movie 3. Figure 2: Time evolution of different kinds of single and double nanobubbles. ( a , b ) The snap shots of TEM images showing the vanishing and stable nanobubbles, respectively. The nanobubbles smaller than critical radius tend to shrink with time and disappear in ~40 s, whereas the larger bubbles persist for more than 10 min. Scale bars, 5 nm. The full movie is available in Supplementary Movie 2 . ( c , d ) The snap shots of TEM images showing the merging of adjacent two nanobubbles observed for 15 and 50 s, respectively. When the nanobubble sizes are significantly different, it shows an Ostwald ripening-like merging process, whereas the similar-sized bubbles are coalescing as their inter-bubble boundary breaks. Scale bars, 10 nm. The full movie is available in Supplementary Movie 3 . 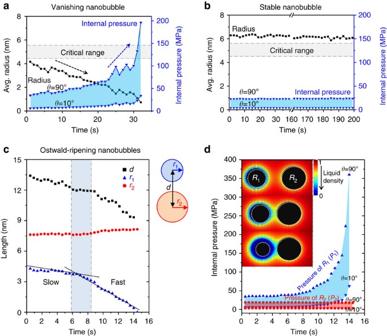Figure 3: Analysis of single nanobubble and Ostwald ripening nanobubbles. (a,b) Average (Avg.) radius and internal pressure changes of vanishing and stable nanobubbles with time, respectively. The pressure was calculated by Young-Laplace equation. The shaded area presents the internal pressure range depending on varying contact angles (θ). (c) Time evolution of radius of growing (red), vanishing (blue) nanobubble and inter-bubble distance measured inFig. 2c. (d) Calculated internal pressure range of Ostwald ripening nanobubbles inFig. 2c. The inset shows the calculation result representing the liquid water density with respect to their relative size and distance between two adjacent nanobubbles, indicating that the water density decreases at the interface region as two bubbles get closer, which is a driving force to put two remote bubbles together. Full size image Figure 3: Analysis of single nanobubble and Ostwald ripening nanobubbles. ( a , b ) Average (Avg.) radius and internal pressure changes of vanishing and stable nanobubbles with time, respectively. The pressure was calculated by Young-Laplace equation. The shaded area presents the internal pressure range depending on varying contact angles ( θ ). ( c ) Time evolution of radius of growing (red), vanishing (blue) nanobubble and inter-bubble distance measured in Fig. 2c . ( d ) Calculated internal pressure range of Ostwald ripening nanobubbles in Fig. 2c . The inset shows the calculation result representing the liquid water density with respect to their relative size and distance between two adjacent nanobubbles, indicating that the water density decreases at the interface region as two bubbles get closer, which is a driving force to put two remote bubbles together. Full size image This result is complementary to those established by the water-ethanol exchange route and AFM. The key differences include that (i) the lateral size of nanobubbles examined by AFM is significantly larger than that shown here, and (ii) the stabilization mechanisms are different. In the AFM studies, it has recently been shown that the interfacial gas enrichment (IGE; interfacial dense gas layer) is the key stabilization mechanism [27] , [28] . The nanobubbles observed here can be stabilized by the mechanism described by the balance between diffusion and attraction of gas molecules to the graphene surface [26] . As our nanobubbles have been prepared by the wet transfer process, the gas concentration at the surface may not be sufficient high to form an IGE, whereas in the water-ethanol exchange the gas concentration at the surface is high and an IGE can be formed. The driving force of the IGE formation is also the attraction between the gas molecules and the solid surface. These different stabilization mechanisms also lead to difference in the contact angles obtained by AFM (~150°) and in here (60–90°). Growth of nanobubbles Nanobubbles are growing by merging with adjacent nanobubbles, which shows clearly different two pathways depending on their relative sizes. In case that the sizes are distinctively different ( R > R ′), the smaller bubble tends to disappear near the surface of the growing larger bubble ( Fig. 2c ), which is similar to Ostwald ripening that is known as a solid-state phenomenon that small crystals are dissolved and redeposited on to the surface of larger crystals. It seems that gas diffuses from one bubble to another across the persisting boundary. On the other hand, two similar-sized nanobubbles ( R ~ R ′) show a coalescing process after breaking their interface, followed by reshaping into dumbbell-like and spherical morphology ( Fig. 2d ). Gas transport between nanobubbles Figure 3a,b shows that there exists critical radius range for the stability of nanobubbles. The nanobubbles whose radii larger than 6 nm persist more than 10 min, whereas smaller bubbles tend to disappear in 1 min. In the Ostwald ripening-like process, the radius of the smaller nanobubble shows a change in slope with respect to time, whereas the radius of the larger bubble steadily increases ( Fig. 3c ). Here, we suppose that a new pathway of gas diffusion is created when the thickness of the interface is smaller than ~2.3 nm, where the instantaneous rupture of the interface allows the massive diffusion from a highly pressurized smaller bubble to a larger bubble. We define it as ‘direct gas diffusion (or transport)’ to be distinguished from ‘indirect gas diffusion’ (see Supplementary Movie 3 ). The internal pressure of the small nanobubble increases from 140 to 400 MPa for the contact angle of 72° as shown in Fig. 3d , which is driving force for gas transport from the small bubble to the large bubble. 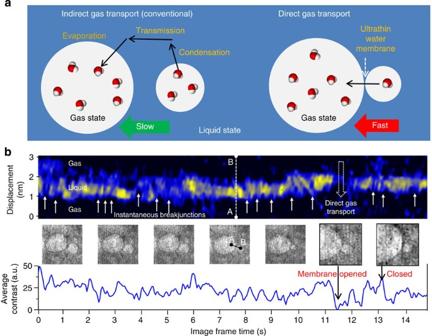Figure 4: Direct and indirect gas transport in Ostwald ripening nanobubbles. (a) Schematic representations explaining indirect and direct gas transport. Between two remote nanobubbles, gases are slowly transported through conventional condensation, transmission and evaporation processes, whereas interfacial nanobubbles show direct gas transport through the ultrathin water membrane without hydration. (b) Time-resolved TEM section analysis of the inter-bubble region (line A-B), extracted fromSupplementary Movie 3. The thickness of water layer gradually decreases with time, and the occurrences of instantaneous breakjunctions are clearly observed as indicated by white arrows. Opening and closing of water membrane are clearly visible between 11 and 13 s. Figure 4 shows the two different pathways of gas transport ( Fig. 4a ) and time-resolved TEM section analysis of Ostwald ripening nanobubbles ( Fig. 4b ). Usually, conventional gas transport between remote nanobubbles includes condensation, transmission and evaporation steps [29] . However, in case that two Ostwald ripening nanobubbles come into contact with each other, the gaseous particles seem to diffuse as a discrete packet from one to another through the ultrathin water membrane without hydration, which needs to be importantly considered for the assembly and function of biomolecules and other systems where nanoscale gas state is involved. The instantaneous breakjunction of the ultrathin water membrane appears dominantly as the thickness decrease below ~2 nm as shown in Fig. 4b . Figure 4: Direct and indirect gas transport in Ostwald ripening nanobubbles. ( a ) Schematic representations explaining indirect and direct gas transport. Between two remote nanobubbles, gases are slowly transported through conventional condensation, transmission and evaporation processes, whereas interfacial nanobubbles show direct gas transport through the ultrathin water membrane without hydration. ( b ) Time-resolved TEM section analysis of the inter-bubble region (line A-B), extracted from Supplementary Movie 3 . The thickness of water layer gradually decreases with time, and the occurrences of instantaneous breakjunctions are clearly observed as indicated by white arrows. Opening and closing of water membrane are clearly visible between 11 and 13 s. Full size image The liquid-phase nanobubbles encapsulated by graphene membrane were visualized by in-situ UHV-TEM, showing the critical radius of nanobubbles determining its long-term stability as well as two different growth processes of merging nanobubbles depending on their relative sizes. It is remarkable that the instantaneous rupture of the ultrathin water membrane between nanobubbles allows direct unhydrated gas transport that has not been observed so far. We believed that this phenomenon needs to be importantly considered in various biological and environmental systems where nanoscale gas state is involved. Other two-dimensional materials such as boron nitride (BN) or molybdenum disulfide (MoS 2 ) are also expected to be useful for the preparation of graphene liquid cells because there might be different behaviours of nanobubbles depending on varying surface hydrophobicity or mechanical flexibility. If additionally mentioned, the exact three-dimensional shape of nanobubble has not been verified experimentally until now. To understand the physical property and the evolution behaviour of nanobubble exactly, it is needed to conduct more in depth study on the side view of nanobubble as a future work. Preparation of monolayer graphene Graphene was synthesized by the chemical vapour deposition method on a high-purity copper foil (Alfa Aesar, 99.999%) with flowing 70 mTorr H 2 and 650 mTorr CH 4 gas. As grown graphene on Cu was spin-coated with poly methyl methacrylate and back-side graphene was etched using oxygen plasma. Then, the poly methyl methacrylate layer on graphene was removed by acetone. Remaining copper was etched in 1.8 wt% ammonium persulfate solution. Finally, the monolayer graphene was rinsed with distilled water several times. HRTEM observation of nanobubbles Electron microscopic analysis was carried out using in-situ UHV-TEM (JEOL, JEM 2010V) operated at 200 keV (refs 12 , 13 ). Its point resolution at Scherzer defocus is 0.23 nm and lattice resolution is 0.20 nm. The ultimate base pressure in the chamber was less than 2 × 10 −10 Torr, and the pressure during observation was below 5 × 10 −9 Torr. All the experiments shown here were performed at room temperature. The UHV in-situ high-resolution TEM (HRTEM) observations were employed optimized parameters for imaging, that is, there were recorded close to the Scherzer defocus and the sample height was adjusted to keep the objects focused in the optimum lens current, because HRTEM images often change depending on the high beam current density and defocus. In-situ real-time HRTEM images were recorded by a digital video recorder at the time resolution of 1/30 s equipped with an online TV camera system (Gatan model 622SC). The typical electron beam current density at the specimens was a very small value of ~1 A cm −2 . It is well known that an electron beam can adversely affect irradiation damages of a sample during examination in an electron microscope (EM; for example, heating, electrostatic charging, ionization damage, displacement damage, sputtering and hydrocarbon contamination) [30] . However, the above-mentioned observation conditions, especially a very small current density and an UHV situation reduced the risk of irradiation damages and hydrocarbon contaminations to the minimum. Although atomic resolution of the JEM 2010V with a LaB6 filament used in this study as compared with that of an EM with a field-emission gun filament falls, its current density is lower by about 100–1,000 times than that of the field-emission gun filament. Moreover, the current density of ~1 A cm −2 at most brings a temperature increase of a few degrees of celsius [30] , which perhaps hardly influences the sample in a recoding time, usually 2–5 min. In fact, while observing the magnified images, no changes in image detail arising from electron beam irradiations were detected. Therefore, we believed that these advantages as well as unique capabilities of graphene liquid cell as a perfect membrane for EM imaging [17] , [31] has enabled the characterization of nanobubbles without contamination in this study. How to cite this article: Shin, D. et al . Growth dynamics and gas transport mechanism of nanobubbles in graphene liquid cells. Nat. Commun. 6:6068 doi: 10.1038/7068 (2015).